An atomic model of brome mosaic virus using direct electron detection and real-space optimization Advances in electron cryo-microscopy have enabled structure determination of macromolecules at near-atomic resolution. However, structure determination, even using de novo methods, remains susceptible to model bias and overfitting. Here we describe a complete workflow for data acquisition, image processing, all-atom modelling and validation of brome mosaic virus, an RNA virus. Data were collected with a direct electron detector in integrating mode and an exposure beyond the traditional radiation damage limit. The final density map has a resolution of 3.8 Å as assessed by two independent data sets and maps. We used the map to derive an all-atom model with a newly implemented real-space optimization protocol. The validity of the model was verified by its match with the density map and a previous model from X-ray crystallography, as well as the internal consistency of models from independent maps. This study demonstrates a practical approach to obtain a rigorously validated atomic resolution electron cryo-microscopy structure. Electron cryo-microscopy (cryo-EM) has progressed to the point of determining near-atomic resolution maps of macromolecular complexes (for example, see refs 1 , 2 , 3 ). However, de novo structure determination remains challenging due to initial model bias, map and model overfitting and/or lack of rigorous map and model validation [4] , [5] . The ultimate goal of a high-resolution cryo-EM study is to derive all-atom models for the macromolecular components of the assembly that pass the rigorous validation metrics routinely applied to X-ray crystallographic structures [6] . This study integrates a number of recently developed technologies, including a direct electron detector, image processing using data beyond conventional radiation damage limits, map validation and resolution assessment using multiple indices, and de novo all-atom modelling, refinement and validation. Using this complete experimental protocol, we report a de novo near-atomic structure of a small (~284 Å in diameter) single-stranded RNA virus, brome mosaic virus (BMV), with a T =3 icosahedral lattice [7] . This designation indicates that there are three quasi-equivalent subunits (QES) in the icosahedral asymmetric unit. A crystal structure is available at a comparable resolution [8] , allowing for subsequent comparison to our results. In addition, its relative small size reduced computational time when testing different image processing protocols. Our goal was to use the crystal structure to post-validate our analysis of the cryo-EM data and to explore whether structural information missing from the crystal structure could be retrieved from the cryo-EM map. Image acquisition using integrating mode with DE-12 Charge-coupled device (CCD) cameras are widely used despite their relatively low signal-to-noise ratio (SNR) at medium to high spatial frequencies [9] , [10] . More recently, the development of radiation-hardened complementary metal-oxide semiconductor (CMOS) detectors that can directly detect primary electrons in an electron microscope has proven a superior alternative to CCD cameras. These new direct detectors have been successfully used for data collection in cryo-EM (for example, see refs 2 , 3 , 11 , 12 ). In addition to improving the spectral SNR (SSNR) of acquired images [12] , [13] , direct detection cameras also provide the advantage of intrinsic dose fractionation by recording multiple images per specimen area within a single continuous exposure (hereafter we refer to this type of data collection as a ‘movie’ and each individual image within the movie a ‘frame’). Frames can be prepared individually or in groups before being used for image reconstruction [2] , [3] , [14] . Direct detection cameras may operate in two different modes: integrating mode or electron counting mode [15] , [16] . Counting mode processes each electron event individually to normalize the energy deposited by each incident electron and/or attempt to more precisely localize each incident electron. This requires a very low exposure per frame and a very high camera frame rate to distinguish individual electron events. Consequently, current implementations of counting mode typically require much longer exposure times than integrating mode [2] , [13] . In contrast, integrating mode generates frames by summing the signal generated by all incident electrons in each pixel without attempting to distinguish each electron event. Therefore, integrating mode is not limited by the beam intensity and the frame rate of the device, and image acquisition can use shorter exposure times to increase throughput and reduce the overall amount of specimen motion due to specimen stage instability. In this study, we used a DE-12 Camera System (Direct Electron, LP), comprised of a 4,096 × 3,072 back-thinned Direct Detection Device (DDD) sensor operated in integrating mode. This camera was installed in the photographic film chamber of a JEM-3200FSC (JEOL, Tokyo, Japan) electron microscope operated at 300 kV with an in-column energy filter (with an energy width of 20 eV). BMV was deposited on a thin continuous carbon substrate (see Methods) to improve the particle distribution and to reduce beam-induced specimen movement. Images were recorded at a nominal microscope magnification of × 50,000, corresponding to a detector magnification of × 60,600. Each movie was collected at 25 frames per second over 1.5 s and a specimen exposure rate of ~35 e − Å −2 s −1 . Therefore, each specimen area was imaged with a cumulative exposure of ~52 e − Å −2 , distributed over 37 frames. This cumulative exposure is 2–3 times the typical number used for high-resolution cryo-EM studies. Various subsets of these frames were used for processing, as described below. Evaluation of particle motion Frame processing methods can be done in two ways: (1) aligning individual or groups of frames or boxed particles from those frames before summing to compensate for specimen motion and/or charging during the course of data recording [2] , [3] , [14] , and/or (2) summing various combinations of frames to generate different particle images used separately for particle orientation determination and for map generation [4] . Here we assess new ways of processing DDD frames to improve the efficiency of image processing and optimize the resolvability of the final reconstruction. Particles were selected using the sum of all frames in a movie (without alignment or other processing procedures), which provided sufficient contrast for particle identification. The particle coordinates were then used to extract the same particle from each of the 37 frames. We then assessed the motion of each of the ~30,000 selected particles throughout their entire 1.5 s exposure. To assess particle motion, we summed three sequential frames for each particle (corresponding to an exposure of 4.2 e − Å −2 ) at different time points within a movie. 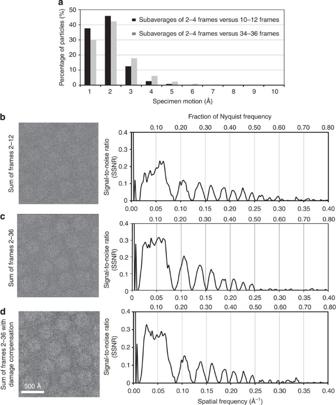Figure 1: Assessment of particle movement and SSNR through the use of movie frames. (a) Histogram showing particle movements assessed by comparing three-frame averages from the beginning, middle and end of each movie. The cumulative exposure was ~53 e−Å−2accumulated over 1.5 s. (b) Left, a magnified portion of a summed frame (2–12). Right, the 1D SSNR of 92 BMV particles computed from that frame. (c) Same asb, from summed frames 2–36. (d) Same asc, from summed frames 2–36, with damage compensation for each frame. Figure 1a shows a histogram of the observed translational shift of the ~30,000 particle data set, between the initial time point (frames 2–4) and either an intermediate time point (frames 10–12) or the ending time point (frames 34–36). The particle motion we observed was relatively small, with only ~1.5 Å mean deviation between the initial and middle time points, and ~2.1 Å mean deviation between the initial and ending time points. Only ~8% of the particles were observed to move >3.3 Å (which corresponded to the resolution of our final density map averaged from the subunits in an asymmetric unit, see detail below) over the entire exposure. This differs from previous reports observed substantial motion, requiring computational motion correction for single particle reconstruction at similar resolution [2] , [3] , [14] . One possible explanation for the observed specimen stability in our data was the use of a continuous carbon support film, which may provide mechanical stability and/or minimize charging by increasing the specimen’s electrical conductivity [17] . Since the detected motion was relatively small (approximately equivalent to the reciprocal of the Nyquist frequency of the imaging conditions), we did not include motion correction in subsequent image processing. Figure 1: Assessment of particle movement and SSNR through the use of movie frames. ( a ) Histogram showing particle movements assessed by comparing three-frame averages from the beginning, middle and end of each movie. The cumulative exposure was ~53 e − Å −2 accumulated over 1.5 s. ( b ) Left, a magnified portion of a summed frame (2–12). Right, the 1D SSNR of 92 BMV particles computed from that frame. ( c ) Same as b , from summed frames 2–36. ( d ) Same as c , from summed frames 2–36, with damage compensation for each frame. Full size image Evaluating SSNR in different frame sums Though most of our data did not appear to be affected by significant charging or specimen motion, this does not guarantee the preservation of high-resolution data. Next, we assessed the SSNR by computing the one-dimensional (1D) power spectrum for various sums of frames in a movie. The left panel of Fig. 1b,c shows an example of a portion of the entire frame summed from frames 2–12 and 2–36 respectively, and right panel shows the 1D SSNR from 92 particles (box size 420 × 420 pixels) extracted from the corresponding summed frames. While we did not correct for motion during the exposure, the first two frames (frames 0 and 1) were removed due to slow beam unblanking in our microscope and known initial beam-induced specimen movement and/or charging [2] , [18] . The power spectrum in Fig. 1b used a cumulative exposure on the specimen of ~18 e − Å −2 , which is considered a safe exposure for high-resolution cryo-EM studies [19] , [20] . The left panel of Fig. 1c represents a cumulative exposure on the specimen of ~53 e − Å −2 for the same specimen area as in Fig. 1b . At this increased cumulative exposure, high-resolution features in biological macromolecules are damaged [19] , [20] , [21] . To eliminate this data from the damaged specimen, we applied radiation damage weighted filtering to each frame prior to summing (hereafter called ‘damage compensation’). This is a series of low-pass filters applied to each frame, modelled after the disappearance of the high-resolution features resulting from radiation damage as described previously [19] , [20] . Using this damage compensation method (see Supplementary Methods ), the overall image contrast at low-resolution was enhanced by between a factor of 1.25 to 2, while preserving high-resolution signal ( Fig. 1b–d ). This factor is not linearly related to the number of frames being averaged (see Supplementary Methods and Supplementary Fig. 1 ). 3D reconstructions using various combinations of frame sums Our goal is to produce the structure with the best quality and resolution from direct detection movie-mode data. To this end, we performed multiple reconstructions using various sums of frames and damage compensation. To properly assess the resolution of our final density maps and to further validate our reconstructions, we followed the gold-standard procedure, that is, dividing the entire set of particle data into two separate data subsets prior to further image processing and 3D reconstruction [22] , [23] . Each data subset used an independent initial model generated by starticos of EMAN1 (ref. 24) [24] ( Fig. 2 ), which builds a rough reconstruction from particles close to the five, three and twofold symmetry axes. Multi-path simulated annealing (MPSA) [25] was used to quickly refine the map to 5 Å. MPSA utilizes cross common lines in Fourier space to determine both centre and orientation of a particle image simultaneously. When the independent reconstructions reached a resolution of ~5 Å, we switched to EMAN1 and used a finer particle orientation search ( Supplementary Fig. 2 ). Resolution was estimated by the 0.143 Fourier shell correlation (FSC) criterion between the two independent reconstructions, with an inner mask to remove the RNA, which lacks overall icosahedral symmetry. The mask had a Gaussian profile with a width of 5 Å to avoid the sharp mask-edge effects, which may cause resolution exaggeration. A combined map was then generated from all of the data, and filtered. The size scale of the map was refined during the model optimization process (Methods). All reported resolutions are based on the final adjusted map scale of 0.99 Å pixel −1 . 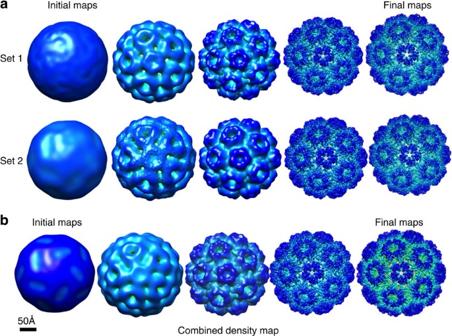Figure 2: Cryo-EM density maps of two independent data sets and 3D reconstructions after 38 refinement iterations. With maps generated from data sets 1 and 2 (a) and their combined maps (b). The initial model for each data set/reconstruction was generated using EMAN1. Subsequent refinement was computed using MPSA. The final five iterations were completed in EMAN1, resulting in the final 3D density maps. Figure 2: Cryo-EM density maps of two independent data sets and 3D reconstructions after 38 refinement iterations. With maps generated from data sets 1 and 2 ( a ) and their combined maps ( b ). The initial model for each data set/reconstruction was generated using EMAN1. Subsequent refinement was computed using MPSA. The final five iterations were completed in EMAN1, resulting in the final 3D density maps. Full size image Particle localization and orientation determination relies heavily on low-resolution signal [26] . Individual frames collected from the DDD camera can be manipulated to optimize low-resolution contrast. We used particle images processed with damage compensation to determine the particle orientations. We then applied these particle orientations to generate different density maps using particle images obtained from various sums of frames. Using the damage-compensated sum of frames 2–36, a map of 3.8 Å resolution was obtained ( Supplementary Fig. 3 ). A similar resolution map was also generated from the sum of frames 2–12 without damage compensation ( Supplementary Fig. 3 ). However, if we used the particle orientations determined solely from the sum of frames 2–12 without damage compensation, the resolution was 4.2 Å. This may be attributable to poorer orientation determination due to relatively low particle contrast. This suggests that the improved contrast from high-exposure, damage-compensated DDD movies yields more accurate particle orientations determination. Additional validation of resolution estimates The gold-standard resolution estimation between two independently determined maps may be influenced by factors including masking, filtering and non-icosahedral symmetry averaging within a complex. To alleviate potential over-refinement that would result in an overly optimistic resolution value, we randomized the phases of the particle data beyond 10 Å, then repeated the refinement procedure. Due to the lack of self-consistent data, a robust refinement procedure should not result in resolution that extends past 10 Å. A significant extension past this resolution is an indication of model bias. This treatment was applied to the two independent data sets, and a sharp fall-off was observed at 10 Å ( Fig. 3a ). According to a recently proposed formula [2] , the ‘True FSC’ is computed from FSC of the original data set and the FSC of the randomized phase data set. The result of this resolution estimation was identical to that from the gold-standard FSC curve between the two independent reconstructions ( Fig. 3a ). 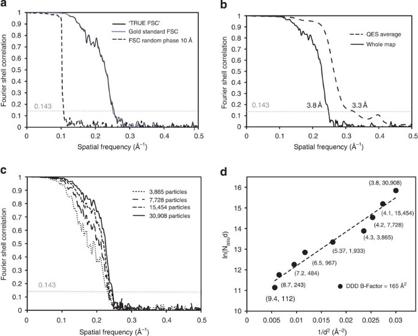Figure 3: Resolution validation of the final cryo-EM density map. (a) FSC curves computed using three different methods (as labelled) between two independent 3D reconstructions generated from two different data sets. (b) Gold-standard FSC curves of the final density maps before and after QES averaging. (c) Gold-standard FSC curves of density maps generated using different total numbers of particles. (d) Relationship between varying number of asymmetric units (equivalent to 60 × total number of particle per reconstruction) and the resolution for each reconstruction as determined inFig. 3c. Each data point refers to the gold-standard resolution and the total number of particles for each reconstruction, respectively. A least-squares linear fit of this relationship resulted in an overallB-factor of 165 Å2. Figure 3: Resolution validation of the final cryo-EM density map. ( a ) FSC curves computed using three different methods (as labelled) between two independent 3D reconstructions generated from two different data sets. ( b ) Gold-standard FSC curves of the final density maps before and after QES averaging. ( c ) Gold-standard FSC curves of density maps generated using different total numbers of particles. ( d ) Relationship between varying number of asymmetric units (equivalent to 60 × total number of particle per reconstruction) and the resolution for each reconstruction as determined in Fig. 3c . Each data point refers to the gold-standard resolution and the total number of particles for each reconstruction, respectively. A least-squares linear fit of this relationship resulted in an overall B- factor of 165 Å 2 . Full size image Estimate of the B -factor of the map Map resolution is dependent on numerous factors including the number of particles (each of which contains 60 asymmetric units in the case of an icosahedral particle such as BMV), specimen or stage motion, envelope functions of the imaging conditions, modulation transfer function of the detector, orientation estimation error and various computational errors throughout the reconstruction steps [25] , [27] , [28] . The cumulative effect of all of these factors can be approximated as a Gaussian function, where the fall-off of Fourier intensity, as a function of resolution, is related to the number of asymmetric units and the ‘ B- factor’ [27] . The B- factor is an excellent indicator of how much data is needed to achieve a particular resolution in a given experimental and computational setting for a given specimen. The B- factor can be approximated by estimating the resolution (as defined above with two independent maps) of various reconstructions using different subsets of particles from the entire data set ( Fig. 3c ). The observed resolution from various number of particles yielded an overall B- factor for our data of ~165 Å 2 , as determined from the slope of Fig. 3d . Based on this B- factor, a map resolution (with imposed icosahedral symmetry) of 4.5 Å requires only 8,274 icosahedral particles (that is, 496,440 asymmetric units), while a resolution of 3.0 Å would require several orders of magnitude more particles (that is, over two million icosahedral particles). A small shift in B- factor will dramatically alter the number of particles needed to achieve this range of near-atomic resolution under the given experimental conditions and computational protocols. Thus, improvements in instrumentation and/or computational protocols can reduce the overall B- factor, and reconstructions targeting a specific resolution would require fewer particles. The above estimation assumes that the structure of all particles is the same to the targeted resolution limit. If the particles are not conformationally identical, and remain mixed in the reconstruction rather than separated into homogeneous classes, the resolution will not be improved by using more particles. Approach for generating and validating models Obtaining an optimal and validated model from the cryo-EM density map is the ultimate goal of high-resolution structural studies. To be confident in our reconstruction, molecular models and inferences, the gold-standard resolution assessment was taken one step further by using intermediate maps to assess potential structural variation in our data and its impact on molecular models. The gold-standard resolution assessment requires that the entire set of raw data (individual particles) be split in half (directly after particle selection) and refined independently, producing two independent density maps (Map B1 and B2, Supplementary Fig. 2 ). A final map was generated from the combined data (Map B). Models were built independently from each of these three maps to avoid bias. By comparing the variation between the two models that used half the data, we can assess the level of detail we can trust in the final model. This provides insight into the potential uncertainty that occurs during model generation. Segment and average three subunits within an asymmetric unit Since the X-ray crystal structure of BMV has been previously determined [8] , the crystal structure could simply have been fitted into the cryo-EM density we generated. However, to test the de novo molecular modelling protocol and our newly developed real-space optimization procedure ( Supplementary Fig. 4 ), we modelled the structure without reference to the crystal structure. The following steps outline the procedures used to generate three optimized, independent all-atom models in a semi-automated manner with no a priori knowledge of the BMV’s structure. Within one asymmetric unit of BMV ( T =3), there are three quasi-equivalent capsid protein subunits that we segmented using Segger [29] , [30] ( Fig. 4a ), an extension for UCSF Chimera which performs semi-automatic segmentation of maps based on density connectivity. The resolvability of our density maps was such that the interfaces between subunits could be readily observed, and we were able to segment out the three individual subunits within one asymmetric unit. The three segmented QES were then aligned using Foldhunter [31] , which performs an exhaustive rigid-body rotation and translation search of the density. The aligned QES were then averaged to improve the visibility of conserved features in the density map. QES averaging typically results in considerably reduced noise [32] and enhanced subunit connectivity compared with the unaveraged subunits [33] . Thus, the ability to determine the protein fold improves. The FSC between the QES averages of the two independent BMV maps (Map E1 and E2, Supplementary Fig. 2 ) showed that the resolution improved to 3.3 Å ( Fig. 3b ). Although the QES-averaged and low-pass filtered map does not suggest any substantial structural differences among the QES, it facilitates the initial establishment of the chain trace using Pathwalker [34] with improved confidence. To account for this inter-subunit variation, unaveraged density maps were used to derive the final models. 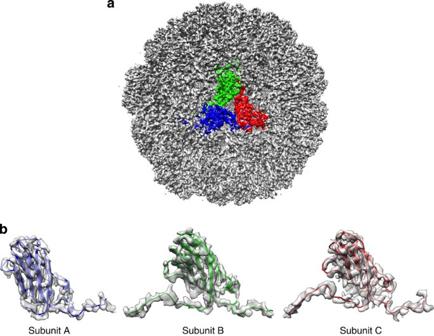Figure 4: Density maps and associated models of segmented subunits in an asymmetric unit. (a) Segmented density of a single asymmetric unit from the final cryo-EM combined density map. Subunit A is blue, subunit B is green and subunit C is red. (b) Final optimized models are displayed with their corresponding segmented density maps. A varying number of amino acids were visible for the terminal arms within each subunit because of disordered regions of density. Figure 4: Density maps and associated models of segmented subunits in an asymmetric unit. ( a ) Segmented density of a single asymmetric unit from the final cryo-EM combined density map. Subunit A is blue, subunit B is green and subunit C is red. ( b ) Final optimized models are displayed with their corresponding segmented density maps. A varying number of amino acids were visible for the terminal arms within each subunit because of disordered regions of density. Full size image De novo Cα models for each subunit map A chain topology from the QES-averaged maps was generated using Pathwalker [8] and a de novo modelling pipeline ( Supplementary Fig. 5 ). Pathwalker populates the density map (Map E, E1 and E2, Supplementary Fig. 2 ) with 164 pseudoatoms (reducing the 189 Cα atoms by 25, due to potentially flexible terminal regions of the capsid subunits) approximating Cα atoms. At this resolution, the density map has β-strand separation and the resulting model matched this density with proper β-sheets. Moreover, both terminal regions could be distinguished in the map and model. Slight manual adjustments were made using Gorgon [35] , an interactive modelling tool designed for building initial models using a density map as a constraint, correcting the Cα–Cα distances generated in Pathwalker. This final model was used as a template to generate the all-atom models for each of the three QES. When placing this template into the three individual subunit maps that together comprised one asymmetric unit, we note that the region including amino acids LYS41-PRO178 (henceforth denoted as the core) was structurally conserved, but that the resolvability of the terminal residues varied for each subunit ( Fig. 4b ). All-atom modelling and real-space optimization Next, we converted our Cα backbone map into an all-atom structure for the core of the capsid using the REMO server [36] . Registration errors (a shift in sequence versus modelled amino acid placement) in amino acid placement were noted based on visible aromatic residue densities, and manually corrected using COOT. N-terminal residues were added for the subunits that had visible density [37] . Each model of the three subunits in the asymmetric unit was optimized in the respective density maps ( Fig. 4b ). To ensure proper fit-to-density, while maintaining good stereochemistry and rotamer assignments, we developed a new real-space optimization routine, called phenix.real_space_refine (underlying implementation described in ref. 38 ) in the Phenix crystallographic software package [39] . Traditionally, Phenix and the other crystallographic packages perform model optimization in reciprocal space, improving the model with respect to X-ray crystallographic data, and thus generating updated phase information for electron density calculations [38] . An alternative approach is to perform the optimization in real space with the aim of improving the model, but not altering the density map as in our case. Real-space refinement has long been used in X-ray crystallography, in particular in the context of interactive model (re)building [37] , [40] , [41] . Advantages include greater control over the refinement and model restraints and rapid local optimization of the model. We combined local real-space model optimization with multiple geometric restraints and automated rotamer fitting to maintain good stereochemistry. Moreover, secondary structure restraints were added to maintain proper distances between β-strands during the refinement stage ( Fig. 4b ). Each round of model optimization was guided by cross-correlation between the map and the model for both the backbone and side chains, independently and in combination ( Supplementary Movie 1 ). In addition, MolProbity (a structure validation tool routinely used in X-ray crystallography) statistics were monitored for proper protein geometry [6] . Additional refinement for regions that had weak density and lacked strong model constraints was performed manually with COOT. Scaling the cryo-EM map pixel After our initial round of model optimization, our density maps were re-calibrated for the map pixel scale and sharpening. In general, precise electron microscope magnification is not as critical for low-resolution as for high-resolution studies for generating accurate atomic model. In practice, the pixel scaling of the final map can be refined during the model-building step. For instance, the pitch of an α-helix may be used to obtain a proper map pixel scale by maintaining correct geometry and having good fit-to-density. Unfortunately, BMV is primarily composed of β-sheets with no α-helices of sufficient length for map pixel calibration. We generated our initial de novo model using the computed map scale value of 0.93 Å pixel −1 from the initial magnification calibration using graphitized carbon. Using this scaling to optimize a larger complex (asymmetric unit as described in the subsequent step) caused fitting errors, and resulted in models that lacked proper polypeptide geometry. When analyzing MolProbity scores, our resulting models had high clash and poor Ramachandran scores. One possible cause was that our initial map pixel scale was inaccurate. We therefore adjusted the map pixel scaling based on model scores, using scales from 0.93 to 1.06 Å pixel −1 while optimizing our all-atom de novo model for each scale. Clash scores and the Ramachandran plot were assessed for each optimized model at the varying scales. The best models resulted when the density map was scaled to 0.99 Å pixel −1 . Obviously, we could have scaled the magnification of our cryo-EM map using the crystal structure. We chose not to do so because the purpose of this investigation was to work out the computational protocol for a specimen having no known crystal structure. However, to validate our scaling procedure, we subsequently did assess the cross-correlation between various scaled maps and the crystal structure. Iterating through the previously used pixel scaling of 0.93 to 1.06 Å pixel −1 , we measured the cross-correlation between our density map and a simulated map generated from the crystal structure. Again, the optimal cross-correlation value was obtained at 0.99 Å pixel −1 , confirming that our map pixel scaling protocol was correct. Therefore, the remainder of our model-building and resolution assessments (as reported in Fig. 3 and Supplementary Fig. 3a ) was then performed using 0.99 Å pixel −1 . All-atom models for asymmetric unit and its neighbours Following the real-space model optimization of individual capsid subunits and adjusting map pixel scale as described above, a complete asymmetric unit was assembled ( Supplementary Fig. 4 ). From these models, an additional round of real-space optimization was performed to improve interfaces and eliminate clashes. The asymmetric unit was iteratively modelled using the real-space optimization routine with minor manual adjustments made in COOT. After five rounds of optimization the asymmetric unit model converged to a final asymmetric unit model with MolProbity and clash score statistics in the top 90% for structures at equivalent resolution. At the next level of interactions, the asymmetric unit interfaces, seven surrounding asymmetric units were added to the original asymmetric unit and real-space optimization was performed on this complex ( Supplementary Movie 2 ). After real-space optimization, our model revealed good fit-to-density and ranked high in terms of protein geometry and clash score ( Table 1 ) when compared with models in the Protein Data Bank (PDB) [42] at equivalent resolution. 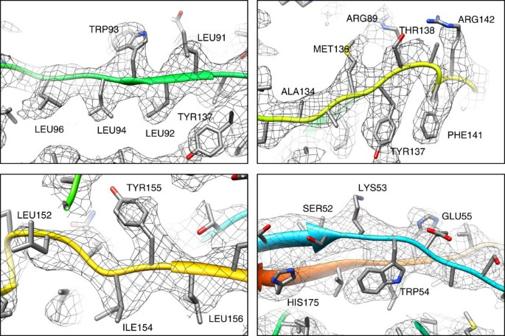Figure 5: Side-chain details from regions in subunit B shown with map and model. Comparable regions from the other two capsid subunits are shown inSupplementary Fig. 5. Figure 5 and Supplementary Fig. 6 show examples of regions of each subunit for their match between density and the model with unambiguous side-chain resolvability. Table 1 MolProbity statistics comparing the cryo-EM map-derived models before and after real space optimization (RSO) and the X-ray structure (PDB id: 1JS9). Full size table Figure 5: Side-chain details from regions in subunit B shown with map and model. Comparable regions from the other two capsid subunits are shown in Supplementary Fig. 5 . Full size image Assessing cryo-EM model and map variation To validate our cryo-EM map and model, we examined the agreement between the two independently optimized models derived from half data sets [43] . The density map and subsequently derived models were optimized from half data sets using the real-space optimization routine ( Fig. 6a ). Variations that exist between the two models may indicate the level of uncertainty for particular regions of the map. Distances between corresponding Cα atoms were computed per residue and, as expected, amino acids with strong density in the backbone and side chains showed little variation. The root mean square deviation (RMSD) between the models generated from maps B1 and B2 ( Fig. 6b ) is 1.96 Å, and no difference in Cα positions was >2.5 Å. This variation in atom placement correlates with potential uncertainty of the models due to weak density. Density at the side-chain level is a key factor in model variation. Obtaining the best fit-to-density at the backbone and side-chain level, while using proper rotamers, resulted in model variation. Well-resolved regions had little variation between the two independently generated models ( Supplementary Fig. 7a ), while poorly resolved regions had greater Cα variation ( Supplementary Fig. 7b ). Amino acids in loops, which are more disordered when compared with β-sheet regions, have higher RMSD values, resulting in a greater level of uncertainty (RMSD of 1.87 Å in β-sheet regions versus 2.10 Å for non β-sheet regions comparing all Cα atoms from the two models). Furthermore, the two data sets have less deviation at the core of the capsid protein (1.51 Å RMSD) when compared with the terminal domains (2.41 Å RMSD), consistent with our comparison of the crystal structure and the cryo-EM model. Finally, a FSC was computed ( Supplementary Fig. 7c ) between the refined model from the even data set (model B1) and the two independent half data set density maps separately. The similarity between the two FSC plots indicate that this model is in agreement with both maps and that overfitting did not occur in the half data sets. 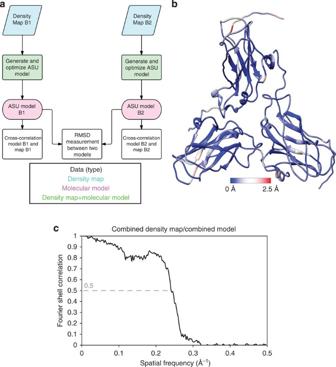Figure 6: Model variation between two independent models derived from the independent data sets. (a) A flow chart outlining the validation procedure used for two independent models. (b) Deviation between the independent models at the Cα level. Blue regions correspond to low deviation between the independent models and red regions correspond to greater deviation. (c) FSC curve between simulated densities generated from the molecular model (after assembling a complete capsid) and the experimental cryo-EM density map. Figure 6: Model variation between two independent models derived from the independent data sets. ( a ) A flow chart outlining the validation procedure used for two independent models. ( b ) Deviation between the independent models at the Cα level. Blue regions correspond to low deviation between the independent models and red regions correspond to greater deviation. ( c ) FSC curve between simulated densities generated from the molecular model (after assembling a complete capsid) and the experimental cryo-EM density map. Full size image Another necessary validation of both the density map and the derived all-atom model is their mutual agreement. As evidenced by the FSC between the combined map and the corresponding model, the two are in agreement up to ~4 Å at 0.5 FSC ( Fig. 6c ). This value is consistent with resolutions computed from the gold-standard resolution assessment and the ‘True FSC’ ( Fig. 3a ). Note, that such a measure is affected by the lack of solvent in the model, which causes a relatively poor agreement at low spatial frequencies relative to conventional FSC curves. Comparison of all-atom models between cryo-EM and crystal We directly compared the quality of our cryo-EM derived model from the combined data set (Map B, Supplementary Fig. 2 ) with the X-ray crystal structure by examining the MolProbity [6] statistical scores ( Table 1 ) and the variation that existed between the two models ( Fig. 7a,b ). The MolProbity results showed that the cryo-EM model was statistically better than the crystal structure. This is likely due to our use of much more rigorous model validation and optimization routines than were available for the crystal structure determination, which was undertaken more than a decade ago [8] . When compared with the crystal structure, our model differs in the more flexible loop regions, and the terminal arms of the subunits. Similar to the crystal structure, subunit A lacked visible density corresponding to the first 40 amino acids at the N-terminal arm, probably attributable to interactions with the disordered RNA [44] . In subunit C, the chain density was traceable from ARG26 in our map ( Fig. 4b ), while the crystal structure was only traced from residue 40. 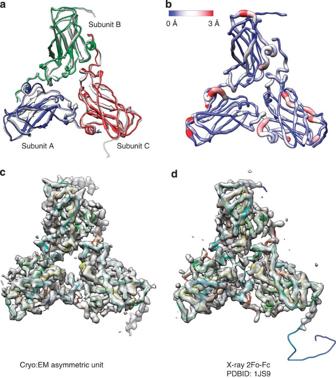Figure 7: Comparisons of cryo-EM and X-ray BMV structures. (a) Overlapping models of cryo-EM (in green, blue and red) and X-ray model (grey, PDB id: 1JS9). (b) Cα deviation between X-ray and cryo-EM derived models. Large deviations are shown in red, with small deviations shown in blue. Cryo-EM map and model (c) and X-ray 2Fo-Fc map (3.55σ) and model (d) of the asymmetric unit. Figure 7: Comparisons of cryo-EM and X-ray BMV structures. ( a ) Overlapping models of cryo-EM (in green, blue and red) and X-ray model (grey, PDB id: 1JS9). ( b ) Cα deviation between X-ray and cryo-EM derived models. Large deviations are shown in red, with small deviations shown in blue. Cryo-EM map and model ( c ) and X-ray 2Fo-Fc map (3.55 σ ) and model ( d ) of the asymmetric unit. Full size image As for the general fold of the capsid protein, our model and the crystal structure are in good agreement ( Fig. 7a ). The Cα RMSD between the cryo-EM model and crystal structure of the asymmetric unit ( Fig. 7b ) was ~1.94 Å (for all amino acids modelled in both structure). In particular, secondary structure elements had less deviation (1.40 Å RMSD) than the loops (2.10 Å RMSD), and the core of the capsid subunits was generally better conserved (1.68 Å RMSD) compared with the terminal arms (3.08 Å RMSD). These computed RMSD values were expected since terminal residues interacting with RNA were likely variable and loops that are surface-exposed generally had high B- factor values in the crystal structure. We computed the FSC to allow comparison of the cryo-EM density ( Fig. 7c ) to the 2Fo-Fc density map generated from deposited structure factors ( Fig. 7d ). The resolution of the resulting FSC curve was 3.8 Å at 0.5, validating the claimed resolution of our map ( Supplementary Fig. 7d ). The maps exhibit high-resolution features such as β-strand separation and some side chains. Connectivity of the capsid protein, specifically the core, was consistent with weaker density at loops. The number of visible amino acids at the terminal arms is consistent between the two maps, even though a poly-alanine tail was added to the crystal structure [8] . Variation did exist at the asymmetric unit center, where density was observed in the crystal structure corresponding to the presence of a magnesium ion from crystallization conditions [8] . This density was absent in the cryo-EM map. Recent studies have demonstrated the superiority of a direct detection camera when compared with a CCD camera used in single particle cryo-EM [2] , [3] , [11] , [12] . Two distinct detector design strategies (counting mode and integrating mode) are currently in use, and each has advantages and disadvantages. In theory, electron counting provides superior SSNR because it reduces noise [15] , [16] . However, counting mode has several practical disadvantages primarily due to limitations of the current hardware. For example, counting mode requires an extremely low exposure (for example, <0.01 electron per pixel per frame) for optimal performance. At increased exposure, the performance diminishes significantly [13] , due to the inability to distinguish coincident electron events in each frame. Users must balance the exposure rate (which is inversely related to the performance of the camera) with exposure time and overall microscopy throughput. However, an integrating mode detector (for example, DE-12) provides increased data throughput and comparable resolutions. Our results also demonstrate the benefit of using damage compensation for single particle cryo-EM studies of biological macromolecules. Damage compensation not only maintains high-resolution signal, but also increases low-resolution signal by removing high-frequency noise in high-exposure direct detection movies. Using damage-compensated data, we successfully obtained a near-atomic resolution density map. A growing concern in the cryo-EM community has become the validation of both maps and models. In this study, we used two non-identical initial starting maps for each data set to eliminate model bias, and tested with randomized phases beyond 10 Å or both data sets to assure no map over-refinement ( Fig. 3a,b , Supplementary Fig. 2 ). Similar to density map assessment, our derived molecular models also required additional validation procedures to describe both quality and potential uncertainty due to map variability ( Fig. 6 ; Supplementary Figs 4 and 7 ). We generated de novo models from our two independent data sets and the combined data set to provide insight into map variability. Once complete, our models, specifically the higher quality model from the combined data set, could be compared with the crystal structure, providing further validation of our all-atom model ( Fig. 7 ; Supplementary Fig. 7d ). Our results reveal that the model variation between the X-ray crystallography model and the cryo-EM model is similar to the variance between the two models generated from the half data sets ( Figs 6b and 7b ). At the Cα backbone level, the variance between the cryo-EM models was as high as 2.5 Å ( Fig. 6 ). This primarily occurred in two specific locations of the capsid protein: (1) the RNA interacting region in the N-terminal arm and (2) physically flexible areas, such as the loops ( Supplementary Figs 6b and 7d ). These model variations are similar for all three subunits. Neither the cryo-EM nor the X-ray crystallography structure resolved the entire polypeptide chain, likely due to the conformational variability of the N-terminal regions and interaction with the encapsulated RNA. BMV virion preparation BMV was generated by an Agrobacterium-mediated gene delivery system that expresses BMV RNA1, RNA2, and RNA3 in Nicotiana benthamiana plants [44] . BMV virions were purified using a method modified from previous procedure [45] . N. benthamiana were grown at a constant 25 °C, 70–75% humidity and a 16:8 h light/dark cycle. Briefly, N. benthamiana leaves were homogenized in buffer I (250 mM NaOAc, 10 mM MgCl2, pH 4.5), and the supernatants were clarified by a 10 min mixing with 10% chloroform. The supernatant was then layered on a 10% sucrose cushion prepared in buffer I, and centrifuged for 3 h at 28,000 r.p.m. using a Beckman SW32 rotor to pellet the virus. The pellets were dissolved in buffer II (50 mM NaOAc, 10 mM MgCl2, pH 5.2) with 38.5% caesium chloride (w/v) and banded by centrifugation for 20 h at 65,000 r.p.m. using a Beckman TLA110 rotor. The virions were collected from the gradient using a needle and dialyzed with three changes of buffer II and stored at −80 °C until use. Cryo-EM specimen preparation and imaging The specimen was prepared by deposition onto a 400-mesh grid with 1.2-μm-hole size (Quantifoil Micro Tools GmbH, Jena, Germany), which we first coated with a thin continuous carbon support film. Each grid was plunge-frozen in liquid ethane and maintained at liquid nitrogen temperature before and during imaging. A total of 30,908 particles were selected for final refinement from 728 total imaging areas (DDD movies). Analysis of specimen motion in DDD frames To detect the movement between each frame in a movie, we used a script to align any potential translational motion of each particle. In this alignment protocol, we ignored potential translational motion along the direction parallel to the electron beam ( z -direction), as well as any potential particle rotation. To improve the accuracy of alignments, we used a box size twice the diameter for each particle, and we summed the boxed particles of every three consecutive frame for the alignment search. Thus, the translational alignment of the i th frame was based on the sum of frames i -1, i and i +1. For each sum of three consecutive frames, the summed particle image was filtered in Fourier space based on the corresponding dark reference image to reduce possible artifacts from fixed pattern noise, and then downsampled by 5 × . Cross-correlation based alignment was calculated based on the tiltxcorr program in IMOD [46] , using the following options: ‘-RotationAngle 0 -FirstTiltAngle 0 -TiltIncrement 0 -FilterRadius2 0.30 -FilterSigma1 0.01 -FilterSigma2 0.02 -CumulativeCorrelation -Iterate 1 -ReverseOrder.’ Damage compensation for DDD frames Since CMOS-based direct detection cameras provide continuous streaming with negligible dead time between frames, the set of frames acquired with each movie represents an exposure series, where each subsequent frame has an incrementally higher cumulative exposure on the specimen. We therefore applied a Gaussian low-pass filter to the Fourier transform of each individual frame (prior to summing multiple frames). The strength of the filter (Gaussian width) applied to each frame was based on the cumulative exposure of the frame. Previous radiation damage studies have deduced the optimal exposure to maximize the SSNR at each spatial frequency for cryo-EM imaging of frozen-hydrated catalase crystal at liquid nitrogen temperature [47] . To be conservative in filtering our data in this study, we arbitrarily added 30% to the exposures determined for catalase crystal. For example, in catalase crystal imaged at 300 kV, the SSNR at 3 Å is maximized at an exposure of ~14 e − Å −2 . Thus, we applied a low-pass filter with a Gaussian width of 1/3 Å −1 to frame 12 (corresponding to a cumulative exposure of ~14 × 1.3=18 e − Å −2 ). Each subsequent frame was low-pass filtered with increasing strength, according to the spatial frequency optimized at the corresponding cumulative exposure. After all frames from each DDD movie were low-pass filtered according to this procedure, they were summed to generate a single image. In theory, the resulting image had maximized SSNR (with respect to radiation damage) over a broad range of spatial frequencies with a relatively high cumulative exposure. Relationship between sum of frames and SSNR An important assumption built into the mathematical formulation performed during single particle analysis is that SSNR will relate linearly with the number of particles ( N ). When tripling the number of frames, however, we observed only up to a twofold improvement in SSNR ( Fig. 1c,d ). To rationalize this discrepancy, we computed the SSNR individually for three different sums of frames (frames 0–12, 13–24 and 25–36) and then summed the three resulting curves ( Supplementary Fig. 1 ). We found that the SSNR of this ‘incoherent sum’ of SSNR curves is substantially higher than the actual SSNR computed from the sum of all 37 frames. This occurrence is due to the portions of the image considered to be signal versus noise. In single particle analysis, the signal is the information from the particle being reconstructed, and the noise is everything else, including statistical noise, detector noise and scattering of the buffer and substrate. When averaging two different but ostensibly identical particles, this works as expected, and SSNR scales linearly to N . However, in movie-mode imaging, the buffer and carbon film substrate are no longer independent for each particle image frame. Instead of averaging incoherently, with sqrt( N ) statistics, as is the case with detector and statistical noise, they average coherently like the particle. This means that our SSNR of multiple sums of frames is no longer the sum of the SSNR of the individual images as it is in single particle averaging, but now scales as some combination between sqrt( N ) and N . Therefore, the relative contribution from the particles (the desired signal) versus the buffer/substrate (which is included in ‘noise’ in our operational definition of SSNR) does not improve with increasing exposure. Increasing exposure only serves to reduce the relative noise levels of the truly random noise sources in the image (for example, detector and statistical noises). Therefore, the SSNR in our operational definition does not improve with exposure as much as expected because the carbon film and the buffer are not really random noise. Note, however, that this does not impact the single particle processing. That process remains mathematically valid, as the solvent and substrate are different for each particle being averaged, and thus can be effectively treated as noise. Map sharpening Before modelling, our density maps (Map B, B1 and B2, Supplementary Fig. 2 ) were subjected to sharpening as follows: We started with our derived B- factor value, sharpening the map with a value of 165 Å 2 to the reported resolution of 3.8 Å using a B- factor script ( http://grigoriefflab.janelia.org/bfactor ). Furthermore, the density map did not exhibit increased noise. We then sharpened the density map by applying various B- factor values at different resolution ranges, none of which improved the resolvability of the density map, while maintaining or reducing the presence of noise. Accession codes: Cryo-EM maps and models of BMV have been deposited in EMDB under accession code EMD-6000 , and in the Protein Data Bank under accession codes 3J7L , 3J7M and 3J7N . The complete EM data set is available for download through the EMDB Electron Microscopy Pilot Image ARchive (EMPIAR), accession codes 10010 and 10011. This includes both raw micrographs and box coordinates. How to cite this article: Wang, Z. et al. An atomic model of brome mosaic virus using direct electron detection and real-space optimization. Nat. Commun. 5:4808 doi: 10.1038/ncomms5808 (2014).